Photonic polarization gears for ultra-sensitive angular measurements Quantum metrology bears a great promise in enhancing measurement precision, but is unlikely to become practical in the near future. Its concepts can nevertheless inspire classical or hybrid methods of immediate value. Here we demonstrate NOON-like photonic states of m quanta of angular momentum up to m =100, in a setup that acts as a ‘photonic gear’, converting, for each photon, a mechanical rotation of an angle θ into an amplified rotation of the optical polarization by mθ , corresponding to a ‘super-resolving’ Malus’ law. We show that this effect leads to single-photon angular measurements with the same precision of polarization-only quantum strategies with m photons, but robust to photon losses. Moreover, we combine the gear effect with the quantum enhancement due to entanglement, thus exploiting the advantages of both approaches. The high ‘gear ratio’ m boosts the current state of the art of optical non-contact angular measurements by almost two orders of magnitude. The precise estimation of a physical quantity is a relevant problem in many research areas. Classical estimation theory asserts that by repeating an experiment N times, the precision of a measurement, defined by the inverse statistical error of its outcome, can be increased at most by a factor of . In quantum physics, this scaling is known as the standard quantum or shot-noise limit, and it holds for all measurement procedures that do not exploit quantum effects such as entanglement. Remarkably, using certain N -particle entangled states it could be possible to attain a precision that scales as N . This is known as the Heisenberg limit, and is the ultimate bound set by the laws of quantum mechanics [1] . Proof-of-principle demonstrations of these quantum-metrology concepts have been given in recent experiments of optical-phase estimation, magnetic-field sensing and frequency spectroscopy [2] , [3] , [4] , [5] , [6] , [7] , [8] , [9] . In photonic approaches, the optimal measurement strategy typically relies on the preparation of ‘NOON’ states [10] , in which all N photons propagate in one arm or the other of an interferometer. However, the experimental preparation of NOON states with large N is extremely challenging, and to date only N =3, 4 and 5 photonic NOON states have been reported [2] , [3] , [4] , [5] . Moreover, as N grows, N -photon entangled states become increasingly sensitive to losses, as the loss of a single photon is enough to destroy all the phase information [11] . It has been proved that, in the presence of losses or other types of noise, no two-mode quantum state can beat the standard limit by more than just a constant factor in the limit of large N [12] , [13] , [14] , [15] . Here we demonstrate the preparation of single-photon NOON-like quantum states that are superpositions of eigenstates of light with opposite total angular momentum quantum numbers. By total angular momentum, we refer here to the sum of the spin-like angular momentum (SAM), associated with left and right circular polarization states, and of the orbital angular momentum (OAM) that characterizes helical modes of light [16] , [17] . Although SAM can have only two values ± ħ , where ħ is the reduced Planck constant, the OAM per photon can generally be given by lħ , where l is an arbitrarily large positive or negative integer. The SAM–OAM superposition states that we generate involve m = l +1 quanta of angular momentum ħ , oriented either parallel or anti-parallel to the propagation axis of each photon. By exploiting such states in the single-photon regime, mechanical rotations can be measured with a precision scaling as m times the square root of the number of probes used. Such enhanced sensitivity can be seen as resulting from a ‘super-resolving’ interference between the two m -quanta angular momentum orientations appearing in the superposition, analogously to the two arms of the NOON-state interferometers. Notably, in this regime every photon is disentangled from all others and hence the loss of a photon does not affect the overall phase coherence, making the scheme loss-robust. Moreover, the experimental state production and detection are exponentially more efficient than for N -photon entangled states. We notice that algorithms for photonic phase estimation without multi-photon entanglement have already been realized [18] . However, these rely on repeated applications of the unknown phase shift to be measured, and remotely coordinated (between Alice and Bob) adaptive measurements. Furthermore, these approaches are exponentially (in the number of applications) sensitive to losses. Although quantum-inspired, our approach is essentially classical because the enhancement does not come from quantum entanglement but results instead from the rotational sensitivity of large angular momentum eigenmodes. In fact, our photonic gears can operate also in the fully classical regime, as described by coherent states. The sensitivity enhancement for a given mechanical rotation is obtained in the form of an ‘amplified’ rotation of the uniform polarization state of the light, that is the mentioned ‘polarization gears’ effect. Rotation sensors based on OAM have been reported before [19] , [20] , [21] , [22] , [23] , but our approach is qualitatively different from all other OAM-related proposals in that we use SAM–OAM combined states that allow us to ‘read’ the rotation by a simple polarization measurement, thus without introducing the large photon losses arising from diffraction or transmission in the angular masks usually needed to read the OAM state. When inserting the photonic gears between polarizers, we observe a ‘super-resolving’ Malus’ law, reminiscent of the polarization correlations visible with multi-photon quantum states [2] , [3] , but which appears in both the classical light or single photon regimes. In this work, we test our photonic gears in three different regimes: classical intense laser light; the single-photon regime, that we adopt to quantitatively compare the achieved angular sensitivity with the shot-noise and Heisenberg limits; and the quantum regime of entangled photons, in which we demonstrate that the photonic gears can be combined with quantum correlations, leading to different kinds of ‘super-resolving’ rotational correlations between the two measurement stages receiving the two photons. In particular, we produce a quantum state that is metrologically equivalent to a NOON state, leading to a hybrid quantum-classical enhancement of the angular sensitivity. The precision attained in this case scales as mN times the square root of the number of probes used, the m originating from the gear ratio and the N (instead of the classical ) from quantum entanglement. We perform a proof-of-principle demonstration with N =2 and total angular momentum up to 18. Photonic gear concept The key element for our photon state manipulations is the q -plate, a novel liquid crystal (LC) device that efficiently maps pure polarization states into hybrid SAM–OAM states and vice versa [24] , [25] , [26] (see Methods and Supplementary Fig. S1 for details). For a linearly polarized input, the photonic states generated are superpositions of m =2 q ±1 quanta in opposite total angular momentum eigenmodes, where q is an integer or semi-integer ‘topological charge’ characterizing the device. Previous achievements were limited to q -plates with low q (up to 3) [27] . In particular, rotational-invariant states with m =0 ( q =1/2) were recently used to demonstrate alignment-free quantum communication [28] . Here, we introduce a new family of devices with q ranging up to 50, producing angular momentum values as large as m =101. These photonic states can be also classically visualized as space-variant polarization states [29] . When these SAM–OAM superposition states are passed through a second q -plate, they are converted back into pure polarization states with zero OAM and a uniform polarization. However, a relative rotation of the transmitting and reading stages by a given angle θ is converted into a rotation of the light optical polarization by the angle mθ , which in our case can be as high as 101 θ . It is this ‘gear ratio’ m that gives rise to the angular sensitivity enhancement. In the following, we explain in greater detail the photonic gears concept by adopting a quantum language, with the purpose of comparing our sensitivity enhancement with the shot-noise and Heisenberg limits and to allow an easier generalization to the hybrid case in which there is both a classical and a quantum effect. Let us then consider the scenario where a sender Alice and a receiver Bob wish to measure a relative misalignment angle θ between their reference frames around the optical axis (see Fig. 1a ). A classical strategy for this task consists of Alice sending N photons (see Fig. 1b ), each one in state , where | n › x denotes a state of n photons in mode x , with x = H, R or L , representing the horizontal-linear, right- and left-circular polarization modes, respectively. All modes in the vacuum state are omitted for brevity. Bob fixes a polarizer in the H direction in his coordinate system, where the misalignment corresponds to a rotation by - θ of the photons’ state. In turn, the L and R polarization states are eigenstates of rotation, so that in Bob’s frame |Ψ C › becomes . The conditional probability that he detects a photon in the H -polarization (of his reference frame) given that the phase is θ is given by Malus’ law: . By measuring this probability, Alice and Bob can estimate θ . To strengthen their statistics, they repeat the procedure ν times, consuming a total of ν × N photons, and average all the outcomes. 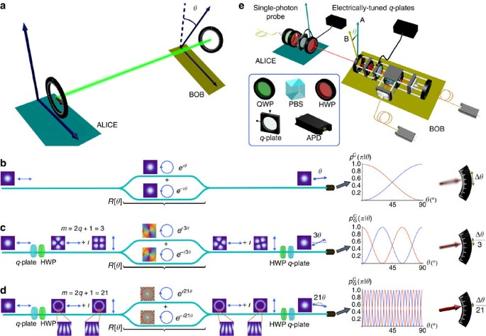Figure 1: Photonic gear concept. (a) A sender Alice prepares and sends to a receiver Bob photonic probes to measure the relative angleθbetween their reference frames. (b–d) Equivalent interferometric scheme. The action of the physical rotation can be schematically represented as an interferometer, where the two arms correspond to the right- and left-circular components of the photon. (b) Polarization-only states are used. The physical rotation introduces a relative phase between the right- and left-circular components of the photon, corresponding to a rotation of the final photon polarization by the same angleθ. The measurement is repeatedνtimes, and polarization fringesare recorded (withπ=H,V), from which the angleθis retrieved with a statistical error Δθ(represented as a blurred arrow pointing to a goniometer). (c–d) Hybrid SAM−OAM photon states are generated by exploitingq-plates [(c)q=1, (d)q=10] and are used to estimate the angleθ. The physical rotation introduces a relative phase between the two components which variesm=2q+1 times faster than the polarization-only case, so that the output photon polarization rotatesmtimes faster (photonic gear effect). The recorded polarization fringesafter decoding with a secondq-plate now present a periodicity∝1/m, leading to an improved angular sensitivity Δθ/m. The intensity (squared blue contour plots) and phase patterns (squared contour plots in false colours) of the linear and circular polarization components of the employed SAM-OAM states are also shown. (e) Experimental setup. In the single-photon regime, Alice uses photons generated by a parametric down-conversion heralded source. In the classical regime, Alice uses coherent laser pulses. The quantum regime, in turn, uses entangled photons and is described inFig. 4. Bob’s detection apparatus is mounted in a compact and robust stage which can be freely rotated around the light propagation axis28. QWP, quarter-wave plate; PBS, polarizing beam-splitter; APD, fibre-coupled single-photon detector. Their final statistical error is bounded as follows: Figure 1: Photonic gear concept. ( a ) A sender Alice prepares and sends to a receiver Bob photonic probes to measure the relative angle θ between their reference frames. ( b – d ) Equivalent interferometric scheme. The action of the physical rotation can be schematically represented as an interferometer, where the two arms correspond to the right- and left-circular components of the photon. ( b ) Polarization-only states are used. The physical rotation introduces a relative phase between the right- and left-circular components of the photon, corresponding to a rotation of the final photon polarization by the same angle θ . The measurement is repeated ν times, and polarization fringes are recorded (with π = H , V ), from which the angle θ is retrieved with a statistical error Δ θ (represented as a blurred arrow pointing to a goniometer). ( c – d ) Hybrid SAM−OAM photon states are generated by exploiting q -plates [( c ) q =1, ( d ) q =10] and are used to estimate the angle θ . The physical rotation introduces a relative phase between the two components which varies m =2 q +1 times faster than the polarization-only case, so that the output photon polarization rotates m times faster (photonic gear effect). The recorded polarization fringes after decoding with a second q -plate now present a periodicity ∝ 1/ m , leading to an improved angular sensitivity Δ θ / m . The intensity (squared blue contour plots) and phase patterns (squared contour plots in false colours) of the linear and circular polarization components of the employed SAM-OAM states are also shown. ( e ) Experimental setup. In the single-photon regime, Alice uses photons generated by a parametric down-conversion heralded source. In the classical regime, Alice uses coherent laser pulses. The quantum regime, in turn, uses entangled photons and is described in Fig. 4 . Bob’s detection apparatus is mounted in a compact and robust stage which can be freely rotated around the light propagation axis [28] . QWP, quarter-wave plate; PBS, polarizing beam-splitter; APD, fibre-coupled single-photon detector. Full size image The right-hand side is the standard quantum limit, and can always be reached in the asymptotic limit of large ν N (ref. 1 ). Our error estimators Δ θ are standard root-mean-squared variances. In general, for phases, a cyclic error cost-function would be more appropriate, as for instance, the Holevo variance [30] . However, both types of variances coincide in the small-error limit, so for our purposes the standard variance is adequate. Using quantum resources, the optimal strategy consists of Alice sending ν probes, each one composed of the N -photon-entangled NOON state . In Bob’s frame, this state is expressed as . The conditional probability that he detects the unrotated state |Ψ Q › is , which resolves values of θ that are N times smaller than p C ( H | θ ). Their uncertainty is then bounded as follows: The right-hand side is now the Heisenberg limit, which can always be reached in the asymptotic limit of large ν (ref. 1 ). In our photonic gear approach, Alice and Bob exchange photons in SAM–OAM superposition states (see Fig. 1c,d ). Alice initially prepares N horizontally polarized photons, as in the classical strategy. However, before sending them to Bob, she first has them pass through a q -plate of charge q . The q -plate implements the bidirectional (unitary) mode transformations , where the subscripts 0 and ±2 q refer to the OAM values, and denotes the creation operator of a photon with polarization π and OAM component l [25] . This results in the following transformation of Alice’s photons: . Next, a half-wave plate (HWP) is used to invert the polarization, to obtain the transmitted states: This single-photon state represents a superposition of m =2 q +1 quanta in opposite total (spin+orbital) angular momentum eigenmodes. Likewise, if the HWP is removed, the case m =2 q −1 is obtained. In Bob’s frame, the photons arrive as . To detect them, he first undoes Alice’s polarization flip with another HWP, and undoes her OAM encoding with another q -plate of the same charge q , so that This state corresponds to a uniform linear polarization, but with the polarization direction forming an angle mθ with respect to Bob’s H axis, resulting in the photonic gear effect. Finally, Bob measures the probability of detecting the H linear polarization conditioned on θ as in the classical strategy. This is again given by Malus’ law: but shows now the m -fold resolution enhancement over the polarization-only strategy. As usual, Alice and Bob repeat the procedure a total of ν times. Their statistical error is now bounded as follows: and can always saturate the bound in the asymptotic limit of large ν N , as shown in Supplementary Note 1 . This represents an improvement over the standard limit (1) for polarization-only strategies by a factor of m . This enhancement is not quantum but due exclusively to the coherent rotational sensitivity of high-order angular momentum eigenmodes. Remarkably, already for the scaling (6) becomes better than the best precision (2) attainable with polarization-only NOON states. Furthermore, the photonic-gear strategies, both in the single-photon and classical regimes, greatly outperform the latter in realistic scenarios with large N . First, the production and detection of our SAM–OAM photon states is exponentially more efficient in N than those of NOON states. Second, as state (3) does not bear any multi-photon coherences, losses reduce the total number of photons, but leave the remaining ones unaltered. That is, total losses characterized by an overall transmissivity 0≤ η ≤1 enter as a constant multiplicative factor, simply rescaling in equation (6) the total number of photons to ν Nη (see Supplementary Note 1 ), in striking contrast to NOON states [11] . Furthermore, one could also consider to exploit the OAM of light to mimic the behaviour of other quantum states such us spin-squeezed states, requiring the superposition of many angular-momentum eigenstates. Combining photonic gears and quantum enhancement The last type of strategy we consider is a hybrid classical-quantum one, which exploits both entanglement and high angular momenta through the photonic gear. In its simplest version, each probe may consist of a N -photon-entangled NOON state . Following the same steps as above, one finds this time that and Thus, ideally, this strategy features the Heisenberg precision scaling for hybrid SAM–OAM approaches, but it bears in practice the same loss-sensitivity problems as the polarization-only quantum strategy. However, for small N , these problems can still be efficiently dealt with and interesting applications can be achieved, as we demonstrate below. Moreover, multi-photon quantum states other than NOON states can also be combined with the photonic gears, obtaining other interesting effects. For example, let us consider two-photon polarization-entangled states, where one photon is sent to Alice and the other to Bob. Alice and Bob make local H / V -polarization analysis in their own rotating stages, which can be set at arbitrary angles θ A and θ B . When θ A = θ B = θ , the system can model two photons travelling in the same mode, subject to the same rotation, and hence yield results analogous to the NOON-state case discussed above for N =2. When θ A ≠ θ B , one can instead align two distant frames remotely with two-photon probes produced by an unrelated common source, which sends one photon to each frame, by exploiting the quantum correlations among the two photons. More in detail, let us assume that the photons are generated in the maximally entangled polarization Bell state . The photons, before transmission, are sent through two q -plates with topological charges q A and q B , respectively, and a HWP, as shown in Fig. 1a . Thus, the following state is distributed to Alice and Bob: Alice and Bob, in their rotated frames, apply the same transformations to the photons, thus converting them back to pure polarization states. The probability that Alice and Bob both detect H -polarized photons in their local frames is then , showing ‘amplified’ polarization correlations. Choosing q A = q B , one can, for example, use these correlations (in combination with classical communication channels) to precisely estimate the relative misalignment θ A – θ B and remotely align the two distant frames. If a HWP with the optical axis parallel to H is now inserted in Bob’s photon path after generation of the polarization-entangled state (which corresponds to acting with a σ x Pauli operator in the R / L basis), one obtains the entangled state , instead of . Alice’s and Bob’s HH -photon correlations have now probability . So, in this case, for θ A = θ B = θ , the system is metrologically equivalent to NOON-state probes for N =2 and . In particular, for N =2 photons, θ can be estimated from the HH -correlation measurements with just half the efficiency as from , which would require two-photon interference detection. Full efficiency in the estimation process can be recovered by simply registering and considering the four possible two-photon polarization correlations ( HH , HV , VH , VV ), which requires no extra measurements. The same result can be generalized to N -photon entangled states. Experimental single-photon gear enhancement Our theoretical predictions were experimentally tested by exploiting a series of q -plates with increasing charge q . We focus first on the single-photon regime. The experimental setup is shown in Fig. 1e . 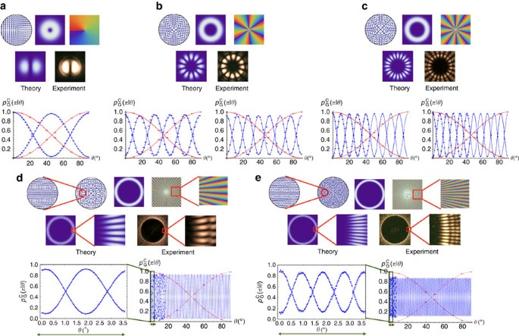Figure 2:Single-photon experimental fringes. Experimental results for single photons andq-plate charges (a)q=1/2 (l=1), (b)q=3 (l=6), (c)q=5 (l=10), (d)q=25 (l=50) and (e)q=50 (l=100). For each case (a−e), we report: theq-plate axis pattern, corresponding to the distribution of the liquid crystal molecular director (top row, left panels); the calculated intensity and phase profiles of the generated OAM fields (top row, middle and right panels); the theoretical and experimental intensities after projection on theH-polarization state (middle panels); the measured fringe patterns (blue dots) as a function of the mechanical rotation angleθ, accompanied by sinusoidal best-fit curves (blue lines) and by the polarization-only case (red dots and lines) (bottom panels). The fringe patterns reported for cases (a,d,e) correspond tom=2q+1 [(a)m=2, (d)m=51 and (e)m=101]. Fringe patterns withm=2q–1 (without the HWPs, left plots) andm=2q+1 (with the HWPs, right plots) are shown in (b) (m=5 and 7) and (c) (m=9 and 11). In (d,e), an inset with a zoomed-in region of the fringes is also shown. Error bars in the polarization fringes are due to the Poissonian statistics of the recorded events, whereas error bars in the set value of the angleθare due to the mechanical resolution of the rotation stage. Figure 2 shows the polarization fringes obtained for several values of q , corresponding to the ‘super-resolving’ Malus’ law (5). The red curves correspond to the polarization-only approach ( q =0), shown for comparison. The oscillation frequency ∝ m =(2 q ±1) highlights the improving angular resolution for increasing q . In Supplementary Fig. S2 , we also show that the initial phase of the oscillation can be tuned by choosing the appropriate input polarization state, and that this allows one in turn to optimize the sensitivity for any angle θ . Figure 2: Single-photon experimental fringes . Experimental results for single photons and q -plate charges ( a ) q =1/2 ( l =1), ( b ) q =3 ( l =6), ( c ) q =5 ( l =10), ( d ) q =25 ( l =50) and ( e ) q =50 ( l =100). For each case ( a − e ), we report: the q -plate axis pattern, corresponding to the distribution of the liquid crystal molecular director (top row, left panels); the calculated intensity and phase profiles of the generated OAM fields (top row, middle and right panels); the theoretical and experimental intensities after projection on the H -polarization state (middle panels); the measured fringe patterns (blue dots) as a function of the mechanical rotation angle θ , accompanied by sinusoidal best-fit curves (blue lines) and by the polarization-only case (red dots and lines) (bottom panels). The fringe patterns reported for cases ( a , d , e ) correspond to m =2 q +1 [( a ) m =2, ( d ) m =51 and ( e ) m =101]. Fringe patterns with m =2 q –1 (without the HWPs, left plots) and m =2 q +1 (with the HWPs, right plots) are shown in ( b ) ( m =5 and 7) and ( c ) ( m =9 and 11). In ( d , e ), an inset with a zoomed-in region of the fringes is also shown. Error bars in the polarization fringes are due to the Poissonian statistics of the recorded events, whereas error bars in the set value of the angle θ are due to the mechanical resolution of the rotation stage. Full size image Experimental imperfections lead to a non-unitary fringe visibility. As shown in Supplementary Note 1 , the loss of visibility increases the statistical error as follows: where V m is the visibility of the oscillation pattern and η m the efficiency of the detection system. In our case, all curves show a visibility greater than 0.73. As a figure of merit for the enhancement in precision, we consider the ratio between the statistical error of the polarization-only strategy and of the photonic gear: . 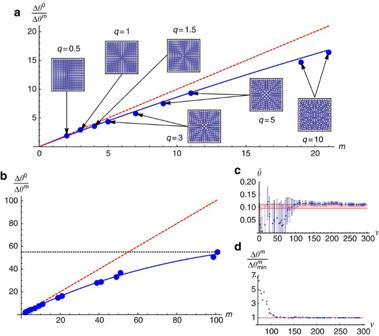Figure 3: Estimation of a rotation angle with photonic gears in the single-photon regime. Ratio between the statistical errors Δθ0/Δθmfor the polarization-only strategy versus the gears strategy in the single-photon regime forq<10 (a) and for all the implemented values ofq(b). In (a) for each point the pattern of the correspondingq-plate is also shown. We obtain a maximum precision enhancement of ≈55 forq=50, corresponding to the generation of optical states with an OAM component withl=100. Red dashed line: theoretical prediction for the ideal case. Blue solid line: model taking into account experimental imperfections (see equation (9) andSupplementary Note 1for more details). Black horizontal dashed line: experimental maximum enhancement. (c,d) Convergence of the angle estimation procedure as a function of the number of repeated experimentsνform=7 (q=3). (c) Measured angleversus the number of incident single photons ν (the red area corresponds to the true angle set in the apparatus, up to mechanical resolution). Error bars correspond to the statistical error in the estimation process. (d) Ratioshowing the convergence to the Cramér–Rao bound (seeSupplementary Note 1). Figure 3a,b shows Δ θ 0 /Δ θ m as a function of m obtained from the interference curves. We obtain a maximum enhancement over the polarization-only strategy by ≈55. To obtain the same precision Δ θ with the polarization-only classical strategy, one would have to increase the number of trials by a factor of 55 2 =3,025, whereas for the polarization-only quantum NOON-state strategy, one would require entangled states of N ≈55 photons each. As shown in Fig. 3c,d , our estimation protocol gives an estimate which converges to the true value θ in a limited number of trials ν~300, where ν is the number of single photons sent through the system. Furthermore, in Supplementary Fig. S2 and Supplementary Note 2 , we discuss a three-step adaptive protocol which permits efficient and unambiguous estimation of such θ even when it is a completely unknown rotation in the full [0, 2π] interval. Figure 3: Estimation of a rotation angle with photonic gears in the single-photon regime. Ratio between the statistical errors Δ θ 0 /Δ θ m for the polarization-only strategy versus the gears strategy in the single-photon regime for q <10 ( a ) and for all the implemented values of q ( b ). In ( a ) for each point the pattern of the corresponding q -plate is also shown. We obtain a maximum precision enhancement of ≈55 for q =50, corresponding to the generation of optical states with an OAM component with l =100. Red dashed line: theoretical prediction for the ideal case. Blue solid line: model taking into account experimental imperfections (see equation (9) and Supplementary Note 1 for more details). Black horizontal dashed line: experimental maximum enhancement. ( c , d ) Convergence of the angle estimation procedure as a function of the number of repeated experiments ν for m =7 ( q =3). ( c ) Measured angle versus the number of incident single photons ν (the red area corresponds to the true angle set in the apparatus, up to mechanical resolution). Error bars correspond to the statistical error in the estimation process. ( d ) Ratio showing the convergence to the Cramér–Rao bound (see Supplementary Note 1 ). Full size image In Supplementary Fig. S3 , we show that the rotational sensitivity enhancement due to the photonic gears effect can also be achieved in the classical regime with an intense laser, making it immediately applicable to real-world optical measurements, which we will now briefly discuss. There, the most common problem is to perform precise non-contact and/or remote optical measurements of roll angles. These are mechanical rotations of an object around one of its symmetry axes [31] , [32] . Polarization-based methods, essentially relying on the Malus’ law combined with suitable polarization manipulations, are among the most convenient approaches. Depending on the details of the scheme, this typically leads to a sensitivity of about 10 −2 degrees for a dynamical range of 30–360°, or about 10 −4 degrees when restricting the range to ~1°. All these polarization-based methods, irrespective of the details, can be combined with our photonic gear tool without changes. Their sensitivity is therefore predicted to be improved approximately by the factor m × V m , which we have shown can be made larger than 50. For example, the method reported in Liu et al. [31] combined with our photonic-gear enhancement is expected to achieve a maximal sensitivity of 10 −6 degrees, or about 0.01 arcsec. The dynamical range is also reduced by a similar factor, but the full dynamical range can be recovered by the adaptive protocol discussed in Supplementary Note 2 . Experimental photonic gears on two-photon entangled states We consider at last the quantum regime of entangled photons, using the setup shown in Fig. 4a . We demonstrate two-photon entangled states where each photon has a different total angular momentum, m 1 and m 2 , with a maximum of m 1 + m 2 =18. We carried out two types of experiments. In the first, we generated photon pairs in the ‘entangled photonic gear state’ , given in equation (8). We then measured the HH correlations for two different sets of q -plates. The results are reported in Fig. 4b–d as a function of the angles θ A and θ B of Alice’s and Bob’s stages. The enhancement in oscillation frequency in both the θ A and the θ B directions with respect to the polarization-only case is clearly observed and matches our theoretical predictions. Next, we generated the entangled state and rotated the two stages by the same angle θ A = θ B = θ , thus creating a situation analogous to the case of NOON-state probes. The measurement results are shown in Fig. 4d . The hybrid quantum-classical sensitivity enhancement by the factor mN = m A + m B =2 q A +2 q B +2 is clearly observed, confirming again our predictions. In particular, the experimental comparison between the two-photon quantum case with and the single-photon case with shows that in the former case a quantum enhancement by a factor 2 is superimposed to the classical photonic gear effect. 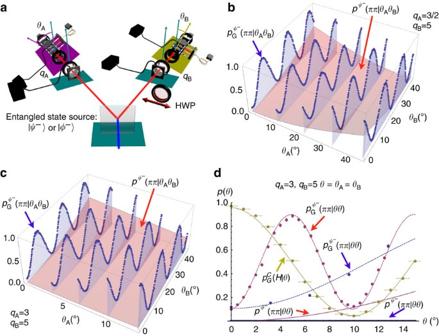Figure 4: Entangled photonic gears. (a) Experimental setup. An entangled photon pair in the polarization state |ψ−› is generated by type-II spontaneous parametric down conversion. The state can be converted to the |−› state by inserting a HWP in the path of Bob’s photon. Each photon is then converted into SAM−OAM hybrid states by theq-platesqAandqBand a HWP, as before, and is sent to a different rotation stage for the analysis. (b) Normalized experimental correlations(blue points), withππ=HH, obtained with the |ψ−› state by measuring the two-fold coincidences in theH-polarization bases on both modes for different values of the rotation anglesθAandθB. We observe the gear enhancement with respect to the polarization-only case (red surface, theory) in the oscillation frequencies in both directionsθA(withmA=2qA−1=2) andθB(withmB=2qB+1=11). (c) Normalized experimental correlations again with |ψ−› (blue points) but formA=2qA+1=7 andmB=2qB+1=11. (d) Normalized experimental correlations obtained with the |ψ−› and |−› states when rotating the two stages by the same angleθA=θB=θ, formA=2qA+1=7 andmB=2qB+1=11. The polarization correlations (blue points: data for |ψ−›, red points: data for |−›) now present an oscillation pattern with a periodicity enhancement of (mA+mB) for |−› andmA–mBfor |ψ−›, due to quantum entanglement combined with the gear effect. The theoretical polarization-onlyHHcorrelation (without the gear enhancement) is also shown, for reference, as a red solid curve in the |−› state case, oscillating as 2θ, and as a blue solid curve in the |ψ−› state case, which is constant and vanishing. Yellow points: experimental data for single-photon gear withm=(mA+mB)/2=9, oscillating at half the frequency of. Dashed curves: best fit of the experimental data. The visibility of the pattern for |−› state is. In all plots, error bars in the correlations are due to the Poissonian statistics of the recorded events, whereas error bars in the set value of the angleθare due to the mechanical resolution of the rotation stage. Figure 4: Entangled photonic gears. ( a ) Experimental setup. An entangled photon pair in the polarization state | ψ − › is generated by type-II spontaneous parametric down conversion. The state can be converted to the | − › state by inserting a HWP in the path of Bob’s photon. Each photon is then converted into SAM−OAM hybrid states by the q -plates q A and q B and a HWP, as before, and is sent to a different rotation stage for the analysis. ( b ) Normalized experimental correlations (blue points), with ππ = HH , obtained with the | ψ − › state by measuring the two-fold coincidences in the H -polarization bases on both modes for different values of the rotation angles θ A and θ B . We observe the gear enhancement with respect to the polarization-only case (red surface, theory) in the oscillation frequencies in both directions θ A (with m A =2 q A −1=2) and θ B (with m B =2 q B +1=11). ( c ) Normalized experimental correlations again with | ψ − › (blue points) but for m A =2 q A +1=7 and m B =2 q B +1=11. ( d ) Normalized experimental correlations obtained with the | ψ − › and | − › states when rotating the two stages by the same angle θ A = θ B = θ , for m A =2 q A +1=7 and m B =2 q B +1=11. The polarization correlations (blue points: data for | ψ − ›, red points: data for | − ›) now present an oscillation pattern with a periodicity enhancement of ( m A + m B ) for | − › and m A – m B for | ψ − ›, due to quantum entanglement combined with the gear effect. The theoretical polarization-only HH correlation (without the gear enhancement) is also shown, for reference, as a red solid curve in the | − › state case, oscillating as 2 θ , and as a blue solid curve in the | ψ − › state case, which is constant and vanishing. Yellow points: experimental data for single-photon gear with m =( m A + m B )/2=9, oscillating at half the frequency of . Dashed curves: best fit of the experimental data. The visibility of the pattern for | − › state is . In all plots, error bars in the correlations are due to the Poissonian statistics of the recorded events, whereas error bars in the set value of the angle θ are due to the mechanical resolution of the rotation stage. Full size image In summary, we have reported a photonic scheme to measure rotation angles with greatly enhanced precision. In the regime of single-photon probes, a precision of has been demonstrated experimentally, with ν N the total number of photons. Notably, rather than in an asymptotic limit, this precision was attained already for total photon numbers as small as ν N ≈10 2 to 10 4 . To our knowledge, this constitutes the highest precision per-particle reported so far [4] , [7] , [9] , [18] . In addition, we demonstrated ultra-sensitive two-photon entangled probes tailored for different target estimations. We anticipate that immediate application of the photonic-gear concept in a classical regime can improve current polarization-based methods for measuring roll angles to a sensitivity of less than 0.01 arcsec. These values provide substantial progress over the current state of the art. In addition to metrological applications, the capability we have demonstrated to efficiently generate and detect hybrid polarization−OAM quantum states with very large OAM creates interesting prospects for high-rate classical communication [33] , coupling with atomic systems [34] , quantum information processing [35] and fundamental tests of quantum mechanics [36] , [37] . Q-plate fabrication A q -plate is essentially a HWP whose optical axis orientation angle is not uniform, but changes from point to point in the transverse plane. The optical axis orientation at each point can be given as θ = q ϕ + α , where θ is the angle the optical axis forms with a reference axis x in the transverse plane xy , ϕ is the azimuthal angle coordinate, q is called the topological charge and α is a constant. When a circularly polarized photon passes through a q -plate, its helicity is switched to the opposite one, like in the case of standard HWPs. Such polarization transformation, although having the same initial and final states, occurs in a different way in different points of the transverse plane, giving rise to a non-uniform geometrical (or Pancharantam−Berry) phase retardation. The phase shift is coordinate dependent and equal to the double of θ , which is equivalent to an OAM state change of ±2 q . The sign of the phase shift depends on the initial polarization state: for the circular |1› L , m input, the output OAM state is changed by +2 q and for the circular |1› R , m one, the output OAM state is changed by −2 q . The same applies to all the superposition states that correspond to an elliptically polarized input photons, producing hybrid SAM–OAM states in the output. This way, with a single q -plate of charge q and linearly polarized Gaussian input it is possible to generate a hybrid state . In our experiment, the q -plates are realized using a nematic LC. A q -plate is a LC cell, in which a thin layer of LC is sandwiched between two glass windows, previously covered with a suitable surface coating for inducing the desired orientational order to the LC layer. For generating the q -plate pattern, we adopted a photoalignment method [38] , which consists in exposing the aligning layer, which contains suitable photosensitive dyes, with linearly polarized UV light. The polarization direction of the light defines the local anisotropy direction of the aligning coating (the latter is actually orthogonal or parallel to the polarization, depending on the choice of materials), which in turn, induces the orientation direction of the LC layer. Hence, the q -plate is realized by illuminating the empty cell with a thin line of light, ‘writing’ sector by sector the desired angular structure, while constantly controlling the polarization direction of the writing beam and rotating the sample at the same time. The LC is inserted in the cell after writing the alignment pattern. The cell glasses also include a thin conducting transparent layer of indium tin oxide, in order to apply an electric field and fine-tune the q -plate to the desired total retardation of half-wave. The output OAM state quality is defined by the smoothness of the q -plate and the size of central defect. The first one is defined by the sample rotation step, laser line thickness and the choice of the aligning surfactant material. The central defect size is also very sensitive to the alignment of the sample with respect to the writing beam. For low topological charges q <10, a step of 1° and corresponding laser line thickness provides good quality of the final structure. With the increase of topological charge, finer q -plate structures required smaller rotation steps (up to 0.1° for q ≥25) and particular attention to rotation error compensation. In combination with suitable azodyes selected as high-resolution aligning surfactants [38] , it was possible to achieve a high quality of the LC alignment and a low size, with respect to the total aligned area, of the central defect. Experimental details The optical source of single photons (not shown) is provided by a Ti:sapphire mode-locked laser, which generates pulses of Δ t =120 fs with repetition rate of 76 MHz at λ =795 nm. The source is then doubled in frequency via a second harmonic generation process to obtain the pump beam of the experiment of λ =397.5 nm and P =700 mW. The single photon is conditionally generated through a type-II spontaneous parametric down conversion process in a l =1.5 mm beta-barium-borate crystal. The output field is then filtered in frequency with a Δ λ =3 mm filter and coupled in a single-mode fibre. Photons at the output of this fibre are then injected into Alice’s preparation device. How to cite this article: D'Ambrosio, V. et al. Photonic polarization gears for ultra-sensitive angular measurements. Nat. Commun. 4:2432 doi: 10.1038/ncomms3432 (2013).